Miz1 is required to maintain autophagic flux Miz1 is a zinc finger protein that regulates the expression of cell cycle inhibitors as part of a complex with Myc. Cell cycle-independent functions of Miz1 are poorly understood. Here we use a Nestin-Cre transgene to delete an essential domain of Miz1 in the central nervous system ( Miz1 Δ POZNes ). Miz1 Δ POZNes mice display cerebellar neurodegeneration characterized by the progressive loss of Purkinje cells. Chromatin immunoprecipitation sequencing and biochemical analyses show that Miz1 activates transcription upon binding to a non-palindromic sequence present in core promoters. Target genes of Miz1 encode regulators of autophagy and proteins involved in vesicular transport that are required for autophagy. Miz1 Δ POZ neuronal progenitors and fibroblasts show reduced autophagic flux. Consistently, polyubiquitinated proteins and p62/Sqtm1 accumulate in the cerebella of Miz1 Δ POZNes mice, characteristic features of defective autophagy. Our data suggest that Miz1 may link cell growth and ribosome biogenesis to the transcriptional regulation of vesicular transport and autophagy. The POZ (Pox virus and Zinc finger) domain/zinc finger protein Miz1 was first identified as a partner protein of Myc and forms a ternary complex with Myc and Max on DNA. Myc/Miz1 complexes block transcription of their target genes in response to specific anti-mitogenic signals; for example, Myc and Miz1 inhibit the activation of the cell cycle inhibitor p15 Ink4b ( Cdkn2b) in response to transforming growth factor-β in tissue culture and in vivo [1] , [2] . Miz1 also forms repressive complexes with Bcl6 and Gfi1; the Bcl6/Miz1 complex represses expression of Cdkn1a and Bcl2 to control proliferation and survival of germinal centre B cells [3] , [4] , [5] . To test the role of Miz1 in vivo , we previously generated mice in which exons that encode the POZ domain of Miz1 are flanked by loxP sites (generating Miz1 Δ POZ mice) [6] , [7] . The Miz1 Δ POZ protein fails to stably associate with chromatin and lacks the ability to regulate gene expression [7] , [8] . Consistent with the biochemical model outlined above, some of the phenotypes observed in Miz1 Δ POZ mice can be explained by complex formation of Myc with Miz1. For example, both Myc and Miz1 are dispensable during normal skin development, but have critical functions during the development of skin papillomas as repressors of Cdkn1a [9] , [10] . In addition, Miz1 has essential functions during early B- and T-cell development that are independent of Myc [7] , [11] , [12] . Specifically, Miz1 is required for the expression of the T-cell receptor β-chain at the cell surface and for interleukin-7-dependent signal transduction [7] , [12] . As Miz1 itself is a DNA-binding protein, one model to explain these findings is that Miz1 binds and directly regulates target genes involved in signal transduction; accordingly, Myc-independent phenotypes might be due to deregulated expression of these genes. Currently, however, neither the DNA sequence to which Miz1 binds nor its direct target genes are known. Miz1 is also highly expressed in many postmitotic cells, including neurons of the peripheral and central nervous systems (CNSs) [13] , arguing that Miz1 function extends beyond regulation of cell proliferation. This prompted us to use a Nestin-Cre strain to delete the POZ domain in the CNS ( Miz1 Δ POZNes ). We report here a genome-wide analysis of Miz1 target genes by ChIP sequencing, gel shift analyses and microarrays that identify Miz1 as a transcriptional regulator of multiple genes involved in vesicular transport, endocytosis and autophagy. Loss of Miz1 function causes cerebellar neurodegeneration To identify roles for Miz1 in neuronal cells, we crossed Miz1 flox/flox mice with mice expressing Cre-recombinase under the control of the Nestin promoter [14] , generating mice that express an amino-terminally truncated protein lacking the POZ domain of Miz1 in the CNS ( Miz1 Δ POZNes ; Supplementary Fig. S1a,b ). Mice of the different genotypes were born at the expected Mendelian frequencies ( Supplementary Fig. S1c ). Analysis of genomic DNA and quantitative reverse transcriptase–PCR (qRT–PCR) experiments confirmed that deletion of exons 3 and 4, which encode the POZ domain, occurred efficiently in the cerebrum, cerebellum, olfactory bulb and, with a lower efficiency, in the eye, which are derived from Nestin-expressing progenitor cells ( Supplementary Fig. S1d,e ). Miz1 Δ POZNes mice initially appeared normal, but were smaller than either wild-type or heterozygous littermates at 5 weeks after birth, and this difference in size increased with age ( Supplementary Fig. S2a ). In addition, Miz1 Δ POZNes mice progressively developed neurological symptoms characterized by slow movement, ataxia and tremor ( Fig. 1a ). As a result, most Miz1 Δ POZNes mice had to be killed at around 18 months of age. Macroscopic analysis revealed that the overall structure of the brain was largely normal in Miz1 Δ POZNes mice, except for the cerebellum. The cerebellum was of normal size in newborn animals, but its relative size decreased over time compared with that of wild-type and heterozygous animals ( Fig. 1b and Supplementary Fig. S2b ). Within the cerebellum, both the white matter and all three layers of the grey matter (Purkinje cells (PCs), molecular layer and granular layer) were reduced in size and appeared disorganized ( Supplementary Fig. S2c ). 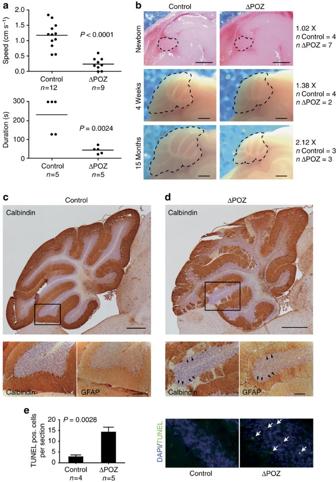Figure 1: Phenotype ofMiz1ΔPOZNesmice. (a)Miz1ΔPOZNesmice move slowly and lack motor coordination. The panel shows the average speed of movement and time on a rotarod (maximum: 300 s) maintained at constant speed of control and age-matchedMiz1ΔPOZNesmice. The average age of mice tested was 16 months.P-values were calculated using an unpaired two-tailed Student’st-test (the number of animals tested is shown below each graph). (b) Defect of cerebellar growth inMiz1ΔPOZNesmice. The panels show sagittal sections of brains of control andMiz1ΔPOZNesmice at the indicated age. Dotted lines show the circumference of the cerebellum. For each mouse, the cerebellar surface area was determined; numbers show the ratio between control andMiz1ΔPOZNesmice. The number of mice analysed for each genotype is indicated on the right. Scale bar, 1 mm. (c,d) Histology of the cerebellum. Sections of the cerebellum of 11-month-old control (c) andMiz1ΔPOZNes(d, please note different scale) mice were stained with antibodies directed against calbindin, a marker for PCs, and glial fibrillary acid protein (GFAP), a marker for Bergman glial cells. Boxes indicate the area of a detail picture in the overviews. GFAP staining is shown for adjacent section (arrowheads: regions of missing PCs). Scale bar, 500 μm (upper panels) and 100 μm (lower panels). (e) Enhanced apoptosis in the granular layer of cerebella inMiz1ΔPOZNesmice. The upper panel shows representative TUNEL (terminal deoxynucleotidyl transferase dUTP nick end labelling) staining of cerebella of age-matched control andMiz1ΔPOZNesmice. The lower panel shows a quantification of staining observed in four control and fiveMiz1ΔPOZNesmice. Error bars show s.e.m.P-value was calculated using an unpaired two-tailed Student’st-test. Figure 1: Phenotype of Miz1 ΔPOZNes mice. ( a ) Miz1 Δ POZNes mice move slowly and lack motor coordination. The panel shows the average speed of movement and time on a rotarod (maximum: 300 s) maintained at constant speed of control and age-matched Miz1 Δ POZNes mice. The average age of mice tested was 16 months. P -values were calculated using an unpaired two-tailed Student’s t -test (the number of animals tested is shown below each graph). ( b ) Defect of cerebellar growth in Miz1 Δ POZNes mice. The panels show sagittal sections of brains of control and Miz1 Δ POZNes mice at the indicated age. Dotted lines show the circumference of the cerebellum. For each mouse, the cerebellar surface area was determined; numbers show the ratio between control and Miz1 Δ POZNes mice. The number of mice analysed for each genotype is indicated on the right. Scale bar, 1 mm. ( c , d ) Histology of the cerebellum. Sections of the cerebellum of 11-month-old control ( c ) and Miz1 Δ POZNes ( d , please note different scale) mice were stained with antibodies directed against calbindin, a marker for PCs, and glial fibrillary acid protein (GFAP), a marker for Bergman glial cells. Boxes indicate the area of a detail picture in the overviews. GFAP staining is shown for adjacent section (arrowheads: regions of missing PCs). Scale bar, 500 μm (upper panels) and 100 μm (lower panels). ( e ) Enhanced apoptosis in the granular layer of cerebella in Miz1 Δ POZNes mice. The upper panel shows representative TUNEL (terminal deoxynucleotidyl transferase dUTP nick end labelling) staining of cerebella of age-matched control and Miz1 Δ POZNes mice. The lower panel shows a quantification of staining observed in four control and five Miz1 Δ POZNes mice. Error bars show s.e.m. P -value was calculated using an unpaired two-tailed Student’s t -test. Full size image Staining of calbindin, a marker for PCs, revealed disruption of the PC layer at 10 months of age and a corresponding increase in Bergmann glia cells as documented by staining with antibodies directed against glial fibrillary acid protein ( Fig. 1c,d ). The PC layer appeared normal at 4 weeks of age, but was largely disrupted at 15 months of age ( Supplementary Fig. S2d ). We also observed increased apoptosis in the granular layer ( Fig. 1e ). This is consistent with observations that the survival of granular neurons depends on synaptic connections with PCs [15] . To understand why Miz1 loss has the strongest effects on PCs, we performed in situ hybridization (ISH) and immunohistochemistry (IHC; Fig. 2a,b ). Both techniques revealed elevated expression of Miz1 mRNA and protein in PCs, suggesting that these cells are particularly sensitive to the lack of a functional Miz1 protein. 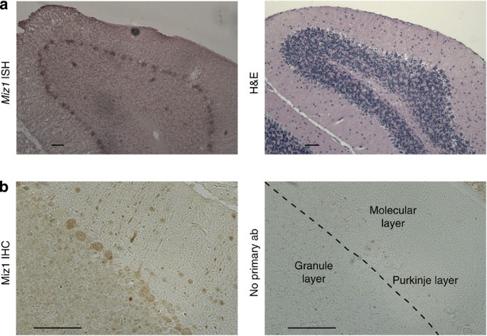Figure 2: Miz1 is highly expressed in PCs. (a) ISH documenting the expression ofMiz1mRNA in PCs of the cerebellum in wild-type mice. Left panel shows ISH, right panel shows haematoxylin and eosin staining. Scale bar, 50 μm. (b) IHC documenting the presence of Miz1 in the nuclei of PCs. The panel on the left shows staining with α Miz1 (H190) antibody, staining on the right is a control staining lacking primary antibody. Scale bar, 50 μm. Figure 2: Miz1 is highly expressed in PCs. ( a ) ISH documenting the expression of Miz1 mRNA in PCs of the cerebellum in wild-type mice. Left panel shows ISH, right panel shows haematoxylin and eosin staining. Scale bar, 50 μm. ( b ) IHC documenting the presence of Miz1 in the nuclei of PCs. The panel on the left shows staining with α Miz1 (H190) antibody, staining on the right is a control staining lacking primary antibody. Scale bar, 50 μm. Full size image Identification of Miz1 target genes and DNA-binding sequence To understand the molecular basis of this phenotype, we identified Miz1 target genes in neuronal cells. We isolated neural progenitor cells from E13.5 brain. After expansion as neurospheres in culture, we performed chromatin immunoprecipitation (ChIP) experiments coupled with high-throughput sequencing to systematically map Miz1-binding sites on chromatin. Statistics for all sequencing experiments are shown in Supplementary Table S1 . This analysis identified 261 sites to which Miz1 bound with high occupancy ( Fig. 3a ; see Supplementary Fig. S3a for more examples and Supplementary Table S2 for a complete list). Control ChIP experiments using independent preparations of chromatin confirmed the specificity of binding ( Supplementary Fig. S3b ). Furthermore, we used a different α-Miz1 antibody and confirmed specific binding of Miz1 to ten on ten sites identified in the genome-wide analysis relative to control regions ( Supplementary Fig. S3c ). The majority of Miz1-binding sites were localized in core promoters close to the transcription start site, unequivocally identifying 140 Miz1-bound promoters (binding site ±1.5 kb of the transcription start site, Fig. 3b ). Comparison with ChIP-sequencing data sets from human mammary epithelial cells (MDA-MB231) showed that binding of Miz1 to these promoters is largely conserved between different cell types and species ( Fig. 3c ; P <5 × 10 −324 using a hypergeometric test). 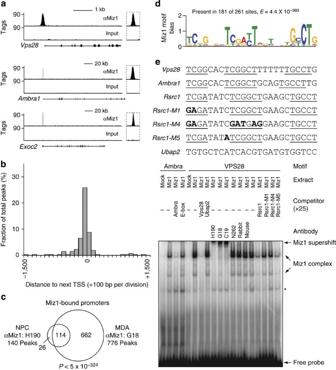Figure 3: Identification of Miz1 target genes and DNA-binding sequence. (a) Representative examples for ChIP-sequencing traces obtained from NPCs using an α-Miz1 antibody. Input traces are shown as negative control. For each gene, the intron/exon structure is shown below the traces with exons indicated as vertical bars and the transcriptional start site (TSS) at the left. An enlarged picture of the peak region is shown on the right. (b) Miz1 binds predominantly to core promoters. The panel shows a histogram of the percentage of promoters with the indicated distances between the peak of the Miz1-binding site and the next TSS. Of all the peaks, 140/261 (54%) are located in core promoters (±1.5 kb). (c) Miz1 binding is conserved across different cell types and species. The plot shows a Venn diagram documenting the overlap in Miz1-bound promoters between murine NPCs and human MDA-MB231 cells (a mammary epithelial tumour cell line). TheP-value was calculated using a hypergeometric test. Note that different α-Miz1 antibodies (H190 and G18) were used for the analysis of mouse and human Miz1-binding sites. (d) Miz1-binding sites contain a conserved sequence element. Sequences (±50 bp) around all 261 Miz1-binding sites observed in NPCs were analysed by MEME-ChIP (‘Motif Analysis of Large DNA Data sets’)16. (e) Electrophoretic mobility shift assay documenting binding of Miz1 to the conserved sequence element (‘Miz1-binding motif’). Nuclear extracts from control HeLa cells (‘Mock’) or cells ectopically expressing Miz1 were incubated with radioactive oligonucleotides spanning the Miz1-binding motif of theAmbra1andVps28promoters. Where indicated, binding reactions included a 25-fold excess of non-labelled oligonucleotides (‘Competitor’), the indicated mutants thereof or of an oligonucleotide containing an E-box sequence from theUbap2promoter. Supershift assays were performed using α-Miz1 (H190, G18 and C19), α-Myc (N262) or control antibodies. *Non-specific band. The sequences of the oligonucleotides used are shown above the panel; mutated nucleotides are shown in bold. Figure 3: Identification of Miz1 target genes and DNA-binding sequence. ( a ) Representative examples for ChIP-sequencing traces obtained from NPCs using an α-Miz1 antibody. Input traces are shown as negative control. For each gene, the intron/exon structure is shown below the traces with exons indicated as vertical bars and the transcriptional start site (TSS) at the left. An enlarged picture of the peak region is shown on the right. ( b ) Miz1 binds predominantly to core promoters. The panel shows a histogram of the percentage of promoters with the indicated distances between the peak of the Miz1-binding site and the next TSS. Of all the peaks, 140/261 (54%) are located in core promoters (±1.5 kb). ( c ) Miz1 binding is conserved across different cell types and species. The plot shows a Venn diagram documenting the overlap in Miz1-bound promoters between murine NPCs and human MDA-MB231 cells (a mammary epithelial tumour cell line). The P -value was calculated using a hypergeometric test. Note that different α-Miz1 antibodies (H190 and G18) were used for the analysis of mouse and human Miz1-binding sites. ( d ) Miz1-binding sites contain a conserved sequence element. Sequences (±50 bp) around all 261 Miz1-binding sites observed in NPCs were analysed by MEME-ChIP (‘Motif Analysis of Large DNA Data sets’) [16] . ( e ) Electrophoretic mobility shift assay documenting binding of Miz1 to the conserved sequence element (‘Miz1-binding motif’). Nuclear extracts from control HeLa cells (‘Mock’) or cells ectopically expressing Miz1 were incubated with radioactive oligonucleotides spanning the Miz1-binding motif of the Ambra1 and Vps28 promoters. Where indicated, binding reactions included a 25-fold excess of non-labelled oligonucleotides (‘Competitor’), the indicated mutants thereof or of an oligonucleotide containing an E-box sequence from the Ubap2 promoter. Supershift assays were performed using α-Miz1 (H190, G18 and C19), α-Myc (N262) or control antibodies. *Non-specific band. The sequences of the oligonucleotides used are shown above the panel; mutated nucleotides are shown in bold. Full size image The binding site for Miz1 on DNA is unknown. To determine whether Miz1 specifically recognizes its target promoters, we used MEME-ChIP (‘Motif Analysis of Large DNA Data Sets’) algorithms to search the ChIP-sequencing data set obtained from neural progenitor cells for conserved sequence motifs in Miz1-bound chromatin. This analysis yielded an extended non-palindromic sequence that is present in the centre of 181 of the 261 Miz1-bound sites ( Fig. 3d ; E =4.4 × 10 −360 ; for definition of E -value, see ref. 16 ). Gel-shift experiments using extracts of HeLa cells ectopically expressing Miz1 identified two complexes that were supershifted with several independent Miz1 antibodies, but not with control or α-Myc antibodies; a weaker, comigrating complex was observed in control cells ( Fig. 3e ). Competition experiments showed that mutation of conserved nucleotides abolished binding to Miz1 to this site, whereas mutation of non-conserved nucleotides did not ( Fig. 3e ). Virtually identical results were obtained with a recombinant Miz1 protein ( Supplementary Fig. S4 ). We concluded that this sequence constitutes a direct binding site for Miz1. To test whether Miz1 activates transcription of it’s target genes, we cloned a 1-kb fragment of the Rorc promoter and oligonucleotides (71 bps) spanning the Miz1-binding site from the Ambra1 promoter, both covering the respective start sites of transcription, in front of a luciferase open-reading frame and performed transient reporter assays. Co-expression of Miz1 stimulated expression of both constructs relative to a control vector, whereas the Miz1 Δ POZ protein was impaired in transactivation ( Fig. 4a ). Similar results had been obtained previously in reporter assays using the Cdkn2b promoter [8] , [17] . Consistent with these results, microarray analyses of RNA isolated from cerebella of wild-type and Miz1 Δ POZNes mice showed that the expression of the 140 genes that are direct targets of Miz1 (see Fig. 3b ) was significantly downregulated in cerebella of Miz1 Δ POZNes mice ( Fig. 4b ). To extend these results, we spiked a gene-set enrichment analysis with a gene set of these Miz1-bound promoters and found that this was the most strongly downregulated and only statistically significant set of genes in this analysis ( Fig. 4c ; P =0.000; false-discovery rate, q =0.002. In this analysis, the nominal P -value is calculated using an empirical phenotype-based permutation test procedure. The q -value (false-discovery rate) is corrected for gene set size and multiple hypothesis testing) [18] . qRT–PCR analyses confirmed that multiple direct target genes of Miz1 were expressed at lower levels in cerebella of Miz1 Δ POZNes mice and that downregulation of Miz1 target genes preceded the appearance of overt pathology, as it was already apparent in phenotypically normal young animals ( Fig. 4d ). In addition, expression of multiple genes specifically expressed in PCs, such as Calbindin , Car8 and Cbln1 , was strongly downregulated in cerebella of 1.5-year-old Miz1 Δ POZNes animals, although these genes were not direct target genes of Miz1, suggesting that their expression was reduced as an indirect consequence due to the loss of PCs. Reduced expression of direct Miz1 target genes was also observed in mouse embryonic fibroblasts isolated from Miz1 Δ POZ mice, demonstrating that Miz1-dependent regulation is not restricted to the cerebellum ( Supplementary Fig. S5a ). Ectopic expression of wild-type Miz1 restored expression of Miz1 target genes ( Supplementary Fig. S5b ). Furthermore, small interfering RNA-mediated depletion of Miz1 decreased expression of Miz1 target genes in mouse embryo fibroblasts (MEFs; Supplementary Fig. S8b ). Finally, IHC as well as immunoblotting confirmed that the protein encoded by one of the Miz1 target genes, Ambra1 , is expressed at lower levels in cerebella and brains of Miz1 Δ POZNes mice relative to wild-type and heterozygous mice ( Supplementary Fig. S5c,d ) and in Miz1 Δ POZ MEFs ( Supplementary Fig. S5e ). Taken together, the data show that Miz1 activates a set of direct target genes in vivo and in tissue culture. 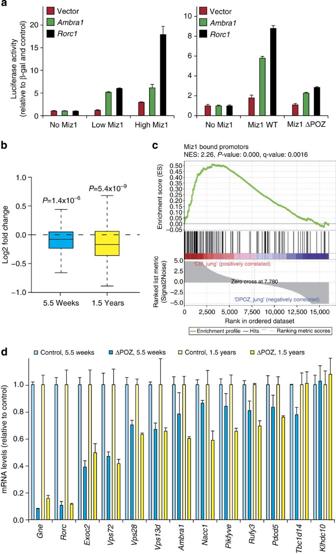Figure 4: Miz1 is a transcriptional activator of genes involved in vesicular transport. (a) Miz1 activates theRorcandAmbra1promoters, and the POZ domain is required for activation. HEK293 cells were transiently transfected with plasmids containing promoter sequences ofAmbra1orRorcin front of luciferase and with expression vectors encoding Miz1 or MizΔPOZ. Empty vectors were used as control. Values were normalized with CMV-βGal. Error bars are s.d. of biological triplicates. (b) Direct target genes of Miz1 are downregulated in cerebella ofMiz1ΔPOZNesmice. Microarray analysis was performed from cerebella of mice at the indicated ages. The panels show box plots (line: median, box: 50% of data points, whisker: 1.5 interquantile range, outliers are not shown) of relative gene expression (plotted as log2-fold change) of the 140 Miz1 direct target genes comparing control andMiz1ΔPOZNesmice. TheP-value was calculated using a Mann–Whitney–Wilcoxon test. Microarrays were performed as technical duplicates from RNA pooled from two animals for each genotype. (c) Gene-set enrichment analysis18documenting significant downregulation of Miz1 target genes in cerebella ofMiz1ΔPOZNesmice.NES, normalized enrichment score. Target genes of Miz1 were the only significant gene set in this analysis. (d) qRT–PCR documenting the expression of selected Miz1 target genes in cerebella of control and ofMiz1ΔPOZNesmice at the indicated ages. Data represent the mean of two independent biological experiments each with three technical replicates. Error bars are s.e.m. Figure 4: Miz1 is a transcriptional activator of genes involved in vesicular transport. ( a ) Miz1 activates the Rorc and Ambra1 promoters, and the POZ domain is required for activation. HEK293 cells were transiently transfected with plasmids containing promoter sequences of Ambra1 or Rorc in front of luciferase and with expression vectors encoding Miz1 or Miz Δ POZ . Empty vectors were used as control. Values were normalized with CMV-βGal. Error bars are s.d. of biological triplicates. ( b ) Direct target genes of Miz1 are downregulated in cerebella of Miz1 Δ POZNes mice. Microarray analysis was performed from cerebella of mice at the indicated ages. The panels show box plots (line: median, box: 50% of data points, whisker: 1.5 interquantile range, outliers are not shown) of relative gene expression (plotted as log 2 -fold change) of the 140 Miz1 direct target genes comparing control and Miz1 Δ POZNes mice. The P -value was calculated using a Mann–Whitney–Wilcoxon test. Microarrays were performed as technical duplicates from RNA pooled from two animals for each genotype. ( c ) Gene-set enrichment analysis [18] documenting significant downregulation of Miz1 target genes in cerebella of Miz1 Δ POZNes mice. NES , normalized enrichment score. Target genes of Miz1 were the only significant gene set in this analysis. ( d ) qRT–PCR documenting the expression of selected Miz1 target genes in cerebella of control and of Miz1 Δ POZNes mice at the indicated ages. Data represent the mean of two independent biological experiments each with three technical replicates. Error bars are s.e.m. Full size image Miz1 target genes are involved in transport and autophagy Neither Ingenuity ( www.ingenuity.com ), gene ontology term, nor gene-set enrichment analysis identified statistically enriched functions or previously identified expression profiles involving Miz1 target genes that could explain the observed phenotype. Functional annotation revealed that multiple target genes of Miz1 encode proteins involved in vesicular transport pathways, endocytosis and lysosomal biogenesis ( Table 1 ). Examples include Vps28, which is involved in sorting ubiquitinated proteins in the endosomal compartment as part of the ESCRT-I complex (endosomal sorting complex required for transport-I) [19] , Exoc2, which is part of the exocyst complex, a multiprotein complex involved in exocytosis and transport from recycling endosomes [20] as well as Pikfyve (Fab1), a phosphatidylinositol kinase that regulates vesicular transport and endocytosis [21] . Endosomal transport and lysosomal biogenesis have been implicated in late steps of autophagy; hence, several target genes of Miz1 involved in vesicular transport have been linked to autophagy ( Table 1 and Supplementary Table S3 ). In addition, several Miz1 target genes encode proteins that have been directly linked to autophagy; examples for this group include Ambra1, an activating cofactor of Beclin1, Gne and Tbc1d14 ( Table 1 ) [22] . Table 1 Functional annotation of selected Miz1 target genes. Full size table As the phenotype of knockout mice that carry brain-specific deletions of the Atg5 or Atg7 genes, which encode E1- and E3-like enzymes for Atg12 conjugation during autophagy, is reminiscent to that of Miz1 Δ POZNes mice, we tested whether Miz1 Δ POZNes mice display phenotypes that might indicate a defective autophagy [23] , [24] . During autophagy, both mono- and polyubiquitinated proteins are sequestered in specific vesicles (‘autophagosomes’) that subsequently fuse with lysosomes, leading to a proteasome-independent degradation of long-lived proteins [25] . We therefore performed IHC with an antibody against ubiquitin and observed a punctate staining in the body of PCs of Miz1 Δ POZNes , but not control mice, arguing that ubiquitinated proteins accumulate in cytoplasmic vesicles or aggregates in these neurons ( Fig. 5a ; for a quantification of staining see Fig. 5d ). In addition, strongly ubiquitin-positive cellular fragments were found in the molecular layer and the white matter of 15-month-old Miz1 Δ POZNes mice, but neither in age-matched control nor in young Miz1 Δ POZNes mice, correlating with the observed phenotypes ( Fig. 5b–d ). Such cellular fragments most likely corresponded to protrusions (dendrites or axons) of cerebellar neurons ( Fig. 5f ). Biochemical fractionation showed that both poly- and monoubiquitinated proteins accumulated in an insoluble form in the cerebella of Miz1 Δ POZNes mice, but not in the brains of control mice, in an age-dependent manner ( Fig. 5e ). Importantly, proteasome activity was identical between cerebella of wild-type and Miz1 Δ POZNes mice, arguing that the accumulation of ubiquitinated proteins was not due to a decrease in proteasome activity ( Supplementary Fig. S6a ). 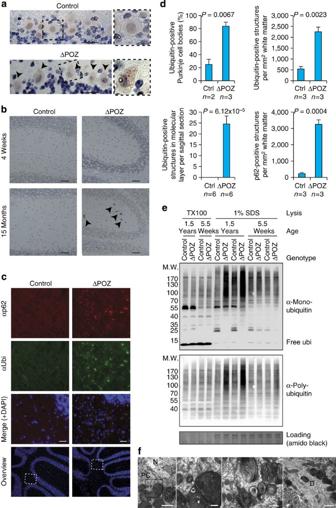Figure 5: Ubiquitinated proteins and p62/Sqstm1 accumulate in an age-dependent manner in cerebella ofMiz1ΔPOZNesmice. (a,b) Immunostaining using an α-ubiquitin antibody of (a) PCs and (b) the molecular layer ofMiz1ΔPOZNesand age-matched control mice (dotted area: higher magnification). Arrowheads designate ubiquitin-positive structures. Scale bar, (a) 25 μm; (b) 50 μm. (c) Immunofluorescence staining using an α-p62 and an α-ubiquitin antibody of the white matter of cerebella fromMiz1ΔPOZNesand age-matched control mice. Nuclei were counterstained with DAPI (4',6-diamidino-2-phenylindole) and overviews of the cerebella clarifying the selected areas are shown. Scale bar, 25 μm. (d) Quantification ofa,bandc. Error bars represent s.e.m. derived from the indicated numbers of animals.P-values were calculated using an unpaired two-tailed Student’st-test. (e) Immunoblots of Triton X-100 soluble (‘TX100’) and insoluble (‘1% SDS’) fractions of cerebella obtained from control andMiz1ΔPOZNesmice of the indicated ages. Blots were probed with antibodies recognizing either mono- or polyubiquitinated proteins. Staining of the membrane with amido black was used as loading control. (f) Transmission electron microscopy documenting the accumulation of large multilamellar bodies in PC bodies (‘PC’) and Purkinje dendrites (‘D’) ofMiz1ΔPOZNesmice (N, nucleus). Such structures were not observed in age-matched control mice (as quantified inSupplementary Fig. S7b). Mean age of mice for all electron microscopy pictures is 13 months forMiz1ΔPOZNesand 12.5 months for control mice. Morphologically similar structures accumulate in neurons of mice deficient in late steps of autophagy28. Scale bars, 2, 0.2, 0.5 and 1 μm, respectively. Figure 5: Ubiquitinated proteins and p62/Sqstm1 accumulate in an age-dependent manner in cerebella of Miz1 ΔPOZNes mice. ( a , b ) Immunostaining using an α-ubiquitin antibody of ( a ) PCs and ( b ) the molecular layer of Miz1 Δ POZNes and age-matched control mice (dotted area: higher magnification). Arrowheads designate ubiquitin-positive structures. Scale bar, ( a ) 25 μm; ( b ) 50 μm. ( c ) Immunofluorescence staining using an α-p62 and an α-ubiquitin antibody of the white matter of cerebella from Miz1 Δ POZNes and age-matched control mice. Nuclei were counterstained with DAPI (4',6-diamidino-2-phenylindole) and overviews of the cerebella clarifying the selected areas are shown. Scale bar, 25 μm. ( d ) Quantification of a , b and c . Error bars represent s.e.m. derived from the indicated numbers of animals. P -values were calculated using an unpaired two-tailed Student’s t -test. ( e ) Immunoblots of Triton X-100 soluble (‘TX100’) and insoluble (‘1% SDS’) fractions of cerebella obtained from control and Miz1 Δ POZNes mice of the indicated ages. Blots were probed with antibodies recognizing either mono- or polyubiquitinated proteins. Staining of the membrane with amido black was used as loading control. ( f ) Transmission electron microscopy documenting the accumulation of large multilamellar bodies in PC bodies (‘PC’) and Purkinje dendrites (‘D’) of Miz1 ΔPOZNes mice (N, nucleus). Such structures were not observed in age-matched control mice (as quantified in Supplementary Fig. S7b ). Mean age of mice for all electron microscopy pictures is 13 months for Miz1 Δ POZNes and 12.5 months for control mice. Morphologically similar structures accumulate in neurons of mice deficient in late steps of autophagy [28] . Scale bars, 2, 0.2, 0.5 and 1 μm, respectively. Full size image Defects in autophagy also cause accumulation of p62/SQSTM1 (ref. 26 ). p62 acts as a receptor for ubiquitinated cargoes and delivers them to the autophagosome; p62 itself is incorporated into the autophagosome and subsequently degraded by autophagy [26] . Cerebella of Miz1 Δ POZNes mice also displayed strongly elevated levels of p62 aggregates, ( Fig. 5c,d ). Notably, ubiquitin-positive structures in the white matter colocalize with p62; virtually identical observations have been reported for other autophagy-deficient strains of mice [27] . Furthermore, p62, similar to the ubiquitinated proteins, accumulated in a detergent-insoluble form ( Supplementary Fig. S6b ). Finally, transmission electron microscopy revealed the accumulation of large polymorphic multilamellar bodies occasionally containing multivesicular or amorphous material in the PC bodies and dendrites of Miz1 Δ POZNes mice ( Fig. 5f and Supplementary Fig. S6c–e ; for a quantification of organelles, see Supplementary Fig. S7b ). These multilamellar bodies are morphologically very similar to membranous cytoplasmic bodies accumulating in autophagy-deficient neurons of Trpml1 (transient receptor potential cation channel/mucolipin1)-deficient animals, expression of which is strongly downregulated in Miz1 Δ POZNes cerebella ( Table 1 ) [28] . Collectively, the findings suggested that PCs in Miz1 Δ POZNes mice had a defect in autophagy that could account for the phenotype of Miz1 Δ POZNes mice. Surprisingly, however, steady-state levels of Lc3/Atg8 that is conjugated to phosphatidylethanolamine (Lc3-II), a marker of autophagy, were unaltered in the cerebella of Miz1 Δ POZNes mice ( Supplementary Fig. S7a ). Furthermore, transmission electron microscopic analysis revealed strong decreases in the number of lysosomes and lipofuscin-containing vesicles, which are thought to be end-stage lysosomes, but did not detect significant changes in the number of autophagosomes ( Supplementary Fig. S7b ). These results either indicate that autophagy is unaltered or that autophagic flux is inhibited at several steps, such that flux is low but no specific intermediates accumulate [29] . Conjugated Lc3 is degraded upon fusion of autophagosomes with lysosomes. Therefore, accumulation of Lc3 in the presence of lysosomal inhibitors can be taken as a measure of autophagic flux allowing us to distinguish between both alternatives [29] . Miz1-dependent autophagic flux To test whether Miz1 is required for maintaining autophagic flux, we isolated primary embryonic fibroblasts from Miz1 flox/flox mice expressing a Cre-ER transgene. Exposure of Miz1 flox/flox Cre-ER + cells to 4-OHT (4-hydroxytamoxifen) induced acute deletion of exons 3 and 4, and decreased the expression of Miz1 target genes ( Fig. 6a,b ). Consistent with the results obtained in vivo , deletion of Miz1 had little effect on Lc3 conjugation in unperturbed cells ( Fig. 6c ). In contrast, the accumulation of conjugated Lc3 that occurs in response to inhibition of lysosomal protein degradation was significantly impaired in Miz1 Δ POZ cells (‘lys PI’ lanes in Fig. 6c ). Addition of 4-OHT had no effect on the expression of Miz1 target genes and autophagic flux in control ( Miz1 flox/flox ) cells ( Fig. 6b,c ), indicating that loss of functional Miz1 impairs autophagic flux. This conclusion is supported by the observation that Miz1 Δ POZ MEFs have a reduced capacity for degradation of long-lived proteins upon amino acid starvation ( Supplementary Fig. S8a ). Notably, deletion of the POZ domain of Miz1 diminished autophagic flux both in normal medium (Dulbecco’s modified Eagle’s medium (DMEM)) and in medium depleted for amino acids (Earle’s balanced salt solution (EBSS)), demonstrating that Miz1 is not required for the induction of autophagy in response to amino acid starvation ( Fig. 6c ). Consistent with this interpretation, expression of Miz1 target genes was decreased in both media ( Fig. 6d ). Furthermore, treatment of MEFs with siRNA targeting Miz1 strongly reduced the expression of multiple target genes of Miz1 involved in membrane traffic and autophagy ( Supplementary Fig. S8b ) and diminished autophagic flux in response to inhibition of lysosomal protein degradation ( Supplementary Fig. S8c ). These observations confirm that the reduction of autophagic flux observed in Miz1 Δ POZ cells is due to loss of Miz1 function. 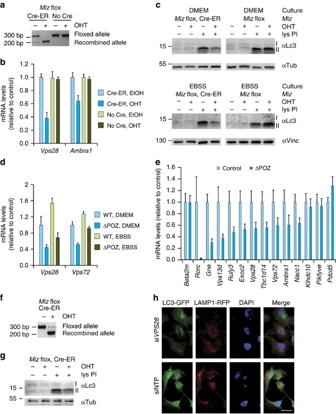Figure 6: Miz1 is required for maintaining autophagic flux. (a) Genomic PCR documenting recombination of the floxedMiz1alleles in Cre-ER-positive and -negative MEFs. 4-OHT was added to the media for 4 days. (b) qRT–PCR assays of Miz1 target genes inMiz1flox/floxCre-ER−andMiz1flox/floxCre-ER+MEFs. The experiment was performed independently from four embryos with identical results. Error bars depict s.d. of technical triplicates from one experiment. (c) Immunoblots using an α-Lc3 antibody detecting Lc3-I and conjugated Lc3-II. 4-OHT-treated and control-treated MEFs of the indicated genotype were incubated with leupeptin and ammonium chloride (lys PI) for 2 h in DMEM (+amino acids) or in EBSS (−amino acids) medium. The expression of α-tubulin (upper panels) or α-vinculin (lower panels) was used as loading control. (d) qRT–PCR assays of Miz1 target genes in control andMiz1ΔPOZMEFs after incubation in DMEM or in EBSS. Error bars depict s.d. of technical triplicates from one experiment. (e) qRT–PCR assays documenting expression of the indicated Miz1 target genes in control andMiz1ΔPOZneurospheres; assays were performed at passage three. s.e.m. values are derived from six biological replicates, each with technical triplicates. (f) Recombination ofMiz1flox/floxCre-ER+neurospheres was tested by genomic PCR. 4-OHT was added to the media for 3 days. (g) Immunoblots using an α-Lc3 antibody detecting Lc3-I and Lc3-II. 4-OHT-treated and non-treatedMiz1flox/floxCre-ER+neurospheres were incubated with leupeptin and ammonium chloride (lys PI) for 30 min. The expression of α-tubulin was used as loading control. (h) Fluorescent microscopy of SHEP cells stably infected with lentiviruses expressing Lc3-GFP and Lamp1-RFP (to mark lysosomes).Vps28was depleted with siRNAs and a non-targeting pool (siNTP) was used as a control. Note the accumulation of Lc3 in vesicles that do not overlap with lysosomes upon depletion of Vps28. Scale bar, 25 μm. Figure 6: Miz1 is required for maintaining autophagic flux. ( a ) Genomic PCR documenting recombination of the floxed Miz1 alleles in Cre-ER-positive and -negative MEFs. 4-OHT was added to the media for 4 days. ( b ) qRT–PCR assays of Miz1 target genes in Miz1 flox/flox Cre-ER − and Miz1 flox/flox Cre-ER + MEFs. The experiment was performed independently from four embryos with identical results. Error bars depict s.d. of technical triplicates from one experiment. ( c ) Immunoblots using an α-Lc3 antibody detecting Lc3-I and conjugated Lc3-II. 4-OHT-treated and control-treated MEFs of the indicated genotype were incubated with leupeptin and ammonium chloride (lys PI) for 2 h in DMEM (+amino acids) or in EBSS (−amino acids) medium. The expression of α-tubulin (upper panels) or α-vinculin (lower panels) was used as loading control. ( d ) qRT–PCR assays of Miz1 target genes in control and Miz1 ΔPOZ MEFs after incubation in DMEM or in EBSS. Error bars depict s.d. of technical triplicates from one experiment. ( e ) qRT–PCR assays documenting expression of the indicated Miz1 target genes in control and Miz1 ΔPOZ neurospheres; assays were performed at passage three. s.e.m. values are derived from six biological replicates, each with technical triplicates. ( f ) Recombination of Miz1 flox/flox Cre-ER + neurospheres was tested by genomic PCR. 4-OHT was added to the media for 3 days. ( g ) Immunoblots using an α-Lc3 antibody detecting Lc3-I and Lc3-II. 4-OHT-treated and non-treated Miz1 flox/flox Cre-ER + neurospheres were incubated with leupeptin and ammonium chloride (lys PI) for 30 min. The expression of α-tubulin was used as loading control. ( h ) Fluorescent microscopy of SHEP cells stably infected with lentiviruses expressing Lc3-GFP and Lamp1-RFP (to mark lysosomes). Vps28 was depleted with siRNAs and a non-targeting pool (siNTP) was used as a control. Note the accumulation of Lc3 in vesicles that do not overlap with lysosomes upon depletion of Vps28. Scale bar, 25 μm. Full size image Consistent with the results obtained in cerebella of Miz1 ΔPOZNes mice, expression of multiple target genes of Miz1 was decreased in cultured neurospheres from E13 embryos of Miz1 Δ POZ and of homozygous Miz1 Δ POZNes mice ( Fig. 6e and Supplementary Fig. S8d ). In contrast, effects on target gene expression were much weaker in heterozygous ( Miz1 flox/wt Cre + ) neurospheres, correlating with the lack of phenotype of these animals ( Supplementary Fig. S8d ). Exposure of neurospheres isolated from Miz1 flox/flox Cre-ER + mice to 4-OHT induced the acute deletion of exons 3 and 4, and diminished autophagic flux as documented by reduced accumulation of conjugated Lc3 in the presence of inhibitors of lysosomal protein degradation ( Fig. 6f,g ). In contrast to the in vivo situation, we failed to detect accumulation of polyubiquitinated proteins in cultured neurospheres ( Supplementary Fig. S8e ). We propose that apoptosis and subsequent cell lysis prevents the detection of polyubiquitinated proteins in cultured Miz1 Δ POZ neurospheres. Consistent with this interpretation, microarray analyses from neurospheres at different passages indicated a progressive reduction in the expression of genes characteristic of neuronal progenitors Miz1 Δ POZ neurospheres in addition to downregulation of Miz1 target genes, suggesting that accumulation of ubiquitinated proteins might lead to the elimination of neuronal progenitors via apoptosis ( Supplementary Table S4 ). Furthermore, transmission electron microscopy revealed the presence of multilamellar bodies in early apoptotic cells found in Miz1 Δ POZ neurospheres ( Supplementary Fig. S8f ). The findings suggested that the lack of changes in steady-state levels of Lc3 conjugation is observed due to blockade of autophagic flux at several steps. Of the Miz1 target genes, Ambra1 is required for autophagosome formation and Lc3 conjugation in mammalian cells [30] . Several members of the ESCRT complex have been implicated in mammalian autophagy, but none of the Miz1 target genes listed in Supplementary Table S2 . We therefore used siRNA to deplete Vps28 in neuroblastoma cells that stably expressed Lc3-GFP and Lamp1-RFP, which marks lysosomes. Upon depletion of Vps28, Lc3 accumulated in vesicles ( Fig. 6h ). Importantly, Lc3 staining did not overlap with staining for the lysosomal marker Lamp1, indicative of a late block in autophagy ( Fig. 6h ). These findings are consistent with observations in Drosophila cells [31] . We concluded that target genes of Miz1 are required at early and late steps of autophagy. We showed here that Miz1 has a critical function in maintaining the viability of PCs in the cerebellum in vivo. In the absence of functional Miz1, cerebella undergo progressive neurodegeneration, which is characterized by an age-dependent accumulation of ubiquitinated proteins and of p62, indicative of defective autophagy. To explain these phenotypes, we used ChIP sequencing to show that Miz1 binds to ~260 target sites in neuronal progenitor cells (NPCs). Target sites of Miz1 had an extended non-palindromic consensus sequence as might be expected for a protein with multiple (13) zinc fingers. Biochemical analysis confirmed that Miz1 directly bound to this sequence. Comparison with data obtained in human mammary epithelial cells (MDA-MB231) showed that these direct target genes were largely conserved between different tissues and species. Miz1-binding sites were predominantly found in core promoters, close to the transcription start site. Reporter assays and comparison with gene expression data showed that Miz1 activates transcription upon binding to its cognate DNA sequence, arguing that the phenotype of Miz1 Δ POZNes mice was due to reduced expression of Miz1 target genes. Comparison with published microarray data showed that the direct Miz1 target genes described here are not subject to regulation by Myc, arguing that their expression may reflect Myc-independent functions of Miz1 ( Supplementary Table S5 ). Defects in distinct cellular processes can lead to accumulation of polyubiquitinated proteins [32] , [33] . One is autophagy and one of the Miz1 target genes described here, Ambra1 , is a bona-fide autophagy gene [30] ; other target genes encode regulators of autophagy (for example, Tbc1d14 and Pdcd5 ; see Supplementary Table S3 for references). Late steps of autophagy involve the fusion of autophagosomes with endosomal vesicles and ultimately lysosomes [22] , [34] . As a result, defects in the progression of endosomes along the endosomal–lysosomal pathway, such as dysfunction of the ESCRT complex proteins, indirectly cause defects in autophagy and accumulation of polyubiquitinated proteins [35] . Multiple proteins encoded by target genes of Miz1 (for example, Vps28 , Pikfyve / Fab1 and Rorc ) were involved in vesicular transport, late steps of autophagosome processing and in fusion of endosomes with lysosomes. We confirmed that depletion of mammalian Vps28 , a direct target gene of Miz1, caused a late block in autophagy. We propose that autophagic flux is reduced in Miz1 Δ POZ cells due to the decreased expression of proteins that act at both early and late stages of the autophagic pathway. This model can explain why steady-state levels of Lc3 conjugation were unaffected by loss of Miz1 in vivo and in cell culture [29] . In postmitotic cells, autophagy is critical for the removal of damaged organelles and toxic protein aggregates; notably, deletion of Atg5 or Atg7 in the CNS has the strongest effect on PCs, similar to what is observed in Miz1 Δ POZNes mice, arguing that survival of these cells is particularly dependent on autophagy [23] , [24] , [36] , [37] . The reduction of autophagic flux observed in Miz1 Δ POZNes mice could therefore account for their progressive neurodegeneration. Notably, the neurodegenerative phenotype of Miz1 Δ POZNes mice is weaker than that of Atg5 or Atg7 knockout mice, most likely due to residual autophagic flux in Miz1 Δ POZNes cells and, by inference, in cerebella of Miz1 Δ POZNes mice. As several target genes of Miz1 encode proteins that are required for intracellular trafficking of multiple cell surface receptors and as regulated transport to the cell surface and endocytosis are critical for the function of the TCR and interleukin-7 receptors that are functionally deficient in Miz1 Δ POZ lymphocytes, we propose that the target genes identified here can also account for other phenotypes observed in Miz1 Δ POZ animals [38] , [39] , [40] , [41] , [42] . Several other transcription factors, such as p53, TFEB and the FoxO family of factors, have been implicated in the transcriptional control of autophagy [43] , [44] , [45] . Notably, there is little overlap in the direct target genes of these factors with those bound by Miz1, suggesting that the precise process within the overall autophagic process that is enhanced by each factor may differ functionally and reflect the specific stimulus or stress response that activates each factor. Previous work had shown that the ribosomal assembly factor, nucleophosmin, is a co-activator of Miz1 (ref. 46 ). In growing cells, nucleophosmin is retained in the nucleolus by the ribosomal protein, Rpl23. Nucleophosmin is released into the nucleolus when Rpl23 levels fall, linking transactivation by Miz1 to defects in ribosome biogenesis. Together with the findings reported here, the data argue that Miz1 is a stress-responsive factor that balances biosynthetic capacity and cell growth with nutrient and energy supply in addition to promoting cell cycle arrest. Mice Miz1 flox/flox and Miz1 +/ Δ POZ mice were crossed to each other and to Nestin-Cre mice [14] to obtain Miz1 Δ POZNes mice. Mice were genotyped by standard PCRs using three different primers listed in Supplementary Table S6 (genomic PCRs). Mice of both sexes between 0 and 18 months (as indicated in figure legends) were used and all mice were included in the analysis. Unless indicated otherwise, mice that carry one or two wild-type alleles of Miz1 and Miz1 flox mice that do not express Nestin-Cre were collectively used as control mice. Speed of movement was measured by placing mice on a grid and determining the distance covered per time. To measure motor coordination, mice were trained for 3 days to the rotarod (Ugo Basile). Subsequently, the time each animal was able to run at a constant speed of 21 r.p.m. was determined. The circumference of the cerebellum was measured and used to estimate surface area. All experiments were carried out according to German law and are approved by an institutional panel (Tierschutzkommission der Regierung von Unterfranken). Immunolabelling and histology All staining were performed on tissue sections collected from OCT- or paraffin-embedded tissues. The following primary antibodies were used: α-Calbindin (1:100; Sigma, C9848), α-glial fibrillary acid protein (OPA1-06100; Pierce), α-Miz1 (1:100, H190; Santa Cruz), α-Ubiquitin (1:100; MBL, MK-11-3) and α-p62 (1:1,000; MBL, pm045). Detection of primary antibodies was carried out with appropriate peroxidase- or fluorochrome-coupled secondary antibodies. Sections were counterstained with haematoxylin. TUNEL (terminal deoxynucleotidyl transferase dUTP nick end labelling) staining was performed using an in situ cell death detection kit (Roche). Klüver–Barrera and haematoxylin and eosin staining was performed according to standard procedures. Pictures were taken with a Leica DM 6000B microscope. Cell culture To isolate NPCs, forebrains of E13.5 Miz1 +/+ , Miz1 Δ POZ or Miz1 flox/flox Cre-ER + embryos were cut in small pieces, digested with trypsin and filtered through sterile gauze. Cells were cultivated in 2:1 DMEM/F12 supplemented with 1 × B27 (Life Technologies), 20 ng ml −1 EGF (Biomol), 20 ng ml −1 basic FGF (Biomol), 1 μg ml −1 fungizone (Gibco) and penicillin/streptomycin (PAA). NPCs were passaged every 7 days. MEFs were isolated from E13.5 Miz1 flox/flox Cre-ER + and Miz1 flox/flox Cre-ER − embryos. To induce recombination in Miz1 flox/flox Cre-ER + NPCs or MEFs, cells were incubated with 200 nM 4-OHT for 3–4 days. Cells were passaged and treated with 20 μM Leupeptin and 20 mM NH 4 Cl for 30 min (NPCs) or 2 h (MEFs) in NPC medium or DMEM and EBSS (MEFs). ChIP assays and parallel sequencing For ChIP assays, cells were cross-linked with 1% formaldehyde at 37 °C for 10 min. Sonication was carried out after swelling in a Bransson sonifier until the majority of fragments showed nucleosomal size. α-Miz1 antibodies (neuronal progenitors: H190; MDA cells: G18 (Santa Cruz)) were coupled to ProteinA/G-Dynabeads (Invitrogen) and used for immunoprecipitation. DNA was purified with Qiagen PCR purification kit after elution of the bound chromatin with 1% SDS and reversion of the crosslink. ChIP DNA was end repaired and A-tailed. Illumina adaptors were ligated to the ChIP DNA fragments. Size fractions (175–225 bp) were cut out from a 1% agarose gel, extracted by Qiagen gel extraction kit and enriched by 18 cycles of PCR amplification. Library size was controlled with the Experion-system (BioRad) and subsequently quantified by picogreen assay and sequenced on an Illumina GAIIx sequencer. Only reads passing the internal Illumina raw data filter were considered. Resulting fastq files were used for alignment to a precompiled reference index (NPCs: mm9, MDA: hg19) with BOWTIE [47] . Peaks were called by MACS [48] using data from the input sample as control and determining a P -value of 10 −10 . GEO accession number for the ChIP-sequencing results is GSE48602 . To compare the Miz1 peaks in NPCs and MDA-MB231 cells, a hypergeometric distribution was used: first the total number of base pairs covered by peaks in each data set was calculated (NPC, 41,500 bp and MDA-MD231, 447,494 bp), and second the number of overlapping base pairs of MDA-MD231 and NPCs peaks was counted (33,176 bp). As population size all murine promoter regions (±1.5 kb around a transcriptional start site; total 93,582,000 bp) were used. Gene expression Total cellular RNA was isolated from whole cerebella or from neurospheres using RNAeasy (Qiagen), including on-column DNA digestion (microarray analysis) or extraction with peqGOLD (Peqlab) for qRT–PCR. For isolation of RNA from the cerebellum, tissue samples were placed into peqGOLD and homogenized with an ultra-turrax. Agilent Mouse Genome Microarray 4 × 44 K v2 was used for the analysis of the gene expression. For qRT–PCR, the first-strand was synthesized with M-MLV Reverse Transcriptase (Invitrogen) and random hexamer primers (Roche). Primer sequences are shown in Supplementary Table S6 . For ISHs, DNA corresponding to exons 3 and 4 of murine Miz1 was cloned into pBluescript KS+ vector and used for synthesis of sense and antisense probe. ArrayExpress accession numbers for the microarray results are E-MEXP-3878 (cerebella) and E-MEXP-3883 (neurospheres). Cell fractionation and immunoblotting Detergent-soluble and -insoluble protein fractions from mouse brains were prepared as described [23] . Briefly, after homogenization, cells were lysed with 0.5% Triton X-100. After centrifugation, the pellet was resuspended in 1% SDS. After SDS–PAGE electrophoresis, proteins were transferred on polyvinylidene difluoride membrane and immunostained for ubiquitinated proteins (07-375; Upstate; MK-11-3, MBL). For immunoblotting of Lc3 in MEFs and NPCs, cells were lysed in buffer containing 50 mM Hepes-KOH, pH 7.5, 150 mM NaCl, 100 mM NaF, 10 mM EDTA and 10 mM Na 4 P 2 O 7 . Immunoblots were probed with antibodies directed against Lc3 (1:1,000; MBL, PM036), α-vinculin (1:10,000; Sigma) and α-tubulin (1:1,000; Chemicon). Full scans of western blots are provided in Supplementary Fig. S9 . Electrophoretic mobility shift assay GST-Miz1 ΔPOZ protein was expressed in Escherichia coli (BL-21) and affinity purified using a glutathione-sepharose (GE Healthcare) column. After elution with glutathione, purity was controlled with a Coomassie Brilliant Blue-stained SDS–PAGE. Dignam nuclear extracts were prepared from HeLa cells transiently transfected with pCDNA3-Miz1. For labelling, 25 pmol of annealed oligonucleotides were labelled using 0.15 mCi γ 32 P-ATP (Hartmann) and 25 U of PNK (NEB), and purified on a G50 column (GE). One microlitre of purified probe was incubated with 2 μl of nuclear extract (~2 mg ml −1 ) in the presence of 20 mM Hepes-KOH, pH 7.9, 10% (v/v) glycerol, 105 mM NaCl, 2 mM MgCl 2 , 50 μM EDTA, 0.25 μg μl −1 salmon sperm DNA, 1.5 mM dithiothreitol, and protease- and phosphatase inhibitors (Sigma) in a 20 μl reaction. For supershifts, 1 μg of antibody was added (Miz1: H190, G18, C19 (all Santa Cruz) Control: rabbit/mouse IgG). After 10 min incubation at room temperature, samples were separated on a 5% PAA-/0.5 × TBE-gel for 5 h at 180 V and exposed on phosphoimager storage screens. Transmission electron microscopy Female mice of different genotypes (three Miz1 Δ POZNes mice and three control mice, 11–15 months of age) were perfusion-fixed in deep anaesthesia via the left ventricle using, after a brief pre-rinse with heparinized saline, 4% paraformaldehyde and 2.5% glutaraldehyde in 0.1 M cacodylate buffer pH 7.3–7.4 (CB). After dissection of the brain and postfixation for at least 18 h, small blocks of the cerebellar tissue were taken from a cerebellar hemisphere of each mouse, washed in CB, osmicated in 2% osmium tetroxide in CB for 2 h, dehydrated in acetone and embedded in Spurr’s medium. Contralateral hemispheres were washed in PBS, cut into coronal 150 μm vibratome sections, osmicated in 1% osmium tetroxide in PBS for 1 h, dehydrated in ethanol and flat-embedded in Epon. Ultrathin sections were contrasted with uranyl acetate and lead citrate and observed in a Leo 912 AB electron microscope (Zeiss NTS, Oberkochen, Germany). Both embedding methods yielded equivalent ultrastructural details for Miz1 Δ POZNes specimens. In situ hybridization Dissected brains were frozen in 2-methylbutane and stored at −80 °C. Serial cryosections (15 μm) were thaw-mounted on microscopic slides, fixed in 4% paraformaldehyde in PBS and stored in 100% ethanol at 4 °C. ISH was carried out using chromogenic detection. Transient transfection assays PCR fragments of the human Ambra1 and Rorc promotor were cloned in a pGL4 plasmid (Clontech). HEK293 cells were transiently transfected (PEI) with the reporter constructs, Miz-WT and Miz Δ POZ expression plasmids and CMV-βgal plasmid. Cells were collected after 48 h, luciferase and β-galactosidase activity was measured according to the manufacturer’s protocol. Endogenous Vps28 protein was depleted in SHEP neuroblastoma cells stably expressing Lc3-GFP [49] and Lamp1-RFP [50] by siRNA (Dharmacon). Long-lived protein degradation assays Degradation of long-lived proteins was measured according to ref. 51 . Cells were labelled with 5 μCi of 35 S-Met/Cys (Hartmann) for 3 h, washed and incubated for 17 h to release short-lived proteins. To block autophagy, cells were partially incubated with 10 mM 3-methyl-adenine (Tocris Bioscience) for 3 h. After another washing, cells were incubated with EBSS or DMEM in the presence/absence of 3-methyl-adenine for 4 h. TCA-cleared supernatant and TCA-washed cells were measured with a scintillation counter. Long-lived protein degradation was calculated by dividing the released radioactivity by total radioactivity. Determination of proteasomal activity Proteasomal activity in cerebella of ΔPOZ and control mice was measured with a Proteasome Activity Assay Kit (Abcam). Fluorescence was measured with a microtitre plate reader (Tecan) in the presence/absence of MG132 after 15 min at 37 °C for 100 min. The MG132-sensitive increase of fluorescence at 350/440 nm was considered as proteasomal activity. Accession codes: ChIP-sequencing data have been deposited in the NCBI Gene Expression Omnibus under accession code GSE48602 . How to cite this article: Wolf, E. et al . Miz1 is required to maintain autophagic flux. Nat. Commun. 4:2535 doi: 10.1038/ncomms3535 (2013).